Sulphur–TiO2yolk–shell nanoarchitecture with internal void space for long-cycle lithium–sulphur batteries Sulphur is an attractive cathode material with a high specific capacity of 1,673 mAh g −1 , but its rapid capacity decay owing to polysulphide dissolution presents a significant technical challenge. Despite much efforts in encapsulating sulphur particles with conducting materials to limit polysulphide dissolution, relatively little emphasis has been placed on dealing with the volumetric expansion of sulphur during lithiation, which will lead to cracking and fracture of the protective shell. Here, we demonstrate the design of a sulphur–TiO 2 yolk–shell nanoarchitecture with internal void space to accommodate the volume expansion of sulphur, resulting in an intact TiO 2 shell to minimize polysulphide dissolution. An initial specific capacity of 1,030 mAh g −1 at 0.5 C and Coulombic efficiency of 98.4% over 1,000 cycles are achieved. Most importantly, the capacity decay after 1,000 cycles is as small as 0.033% per cycle, which represents the best performance for long-cycle lithium–sulphur batteries so far. There has been a steady increase in the demand for high-performance and long-lasting rechargeable batteries for a wide range of applications, ranging from portable electronics and consumer devices to electric vehicles and large-scale grid energy storage [1] , [2] , [3] , [4] , [5] , [6] , [7] , [8] , [9] . Unfortunately, the energy density and cycle life of existing lithium-ion batteries remain insufficient for many of the aforementioned applications, prompting the urgent need for new electrode materials with much higher charge capacities [1] , [2] , [3] , [4] , [5] . Over the years, significant progress has been made in the development of new high-performance anode materials (such as silicon and tin) for rechargeable batteries [10] , [11] , [12] , [13] , [14] , but the major limiting factor is still the relatively low capacity of cathodes. Sulphur is a promising cathode material with a theoretical specific capacity of 1,673 mAh g −1 , which is ~5 times that of existing materials based on transition metal oxides and phosphates [15] , [16] , [17] , [18] . However, many challenges remain in developing a practical lithium–sulphur battery for commercialization. It is known that sulphur particles suffer from the problems of (a) poor electronic conductivity, (b) dissolution of intermediate polysulphides and (c) large volumetric expansion (~80%) upon lithiation, which results in rapid capacity decay and low Coulombic efficiency ( Fig. 1a ) [15] , [16] , [17] , [18] . Over the years, extensive efforts have been devoted to addressing the first two problems, by encapsulating sulphur particles with conducting materials, including porous carbon [19] , [20] , [21] , [22] , [23] , [24] , [25] , [26] , [27] , graphene oxide [28] , [29] and conductive polymers [30] , [31] , [32] , [33] , in an attempt to improve their electronic conductivity and limit polysulphide dissolution. However, insufficient emphasis has been placed on dealing with the third challenge—the large volumetric expansion of sulphur during lithiation coupled with polysulphide dissolution. This poses a critical problem because volume expansion of the sulphur core will cause the protective coating layer to crack and fracture, rendering the conventional core–shell morphology [32] , [33] , [34] , [35] ineffective in trapping polysulphides ( Fig. 1b ). In this respect, the strategy of adjusting the amount of sulphur infusion into mesoporous carbon has been demonstrated [20] , [23] , but it can be difficult to control the uniformity of sulphur filling within the pores of each particle and across different particles. Overall, the long-term cycling performance for lithium–sulphur batteries remains to be improved. 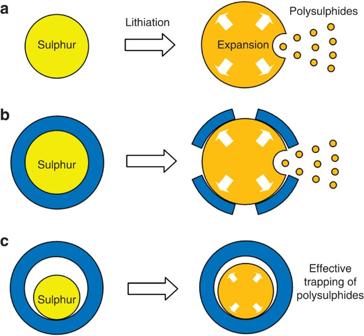Figure 1: Schematic of the lithiation process in various sulphur-based nanostructure morphologies. (a) Bare sulphur particles undergo large volumetric expansion and polysulphide dissolution upon lithiation, resulting in rapid capacity decay and low Coulombic efficiency. (b) Although the core–shell morphology provides a protective coating, cracking of the shell will occur upon volume expansion of sulphur during lithiation, leading to polysulphide dissolution as well. (c) The yolk–shell morphology provides internal void space to accommodate the volume expansion of sulphur during lithiation, resulting in a structurally intact shell for effective trapping of polysulphides. Figure 1: Schematic of the lithiation process in various sulphur-based nanostructure morphologies. ( a ) Bare sulphur particles undergo large volumetric expansion and polysulphide dissolution upon lithiation, resulting in rapid capacity decay and low Coulombic efficiency. ( b ) Although the core–shell morphology provides a protective coating, cracking of the shell will occur upon volume expansion of sulphur during lithiation, leading to polysulphide dissolution as well. ( c ) The yolk–shell morphology provides internal void space to accommodate the volume expansion of sulphur during lithiation, resulting in a structurally intact shell for effective trapping of polysulphides. Full size image Herein, we demonstrate for the first time, the design of a sulphur–TiO 2 yolk–shell nanoarchitecture for stable and prolonged cycling over 1,000 charge/discharge cycles in lithium–sulphur batteries. The unique advantage of the yolk–shell morphology lies in the presence of internal void space to accommodate the large volumetric expansion of sulphur during lithiation, thus preserving the structural integrity of the shell to minimize polysulphide dissolution ( Fig. 1c ). In comparison with bare sulphur and sulphur–TiO 2 core–shell nanoparticles, the yolk–shell nanostructures are found to exhibit the highest capacity retention owing to the effectiveness of the intact TiO 2 shell in limiting polysulphide dissolution. Using the yolk–shell nanoarchitecture, an initial specific capacity of 1,030 mAh g −1 at 0.5 C and Coulombic efficiency of 98.4% over 1,000 cycles is achieved. Most importantly, the capacity decay at the end of 1,000 cycles is found to be as small as 0.033% per cycle (3.3% per 100 cycles). To the best of our knowledge, this is the first time that a lithium–sulphur battery with this level of performance has been described. Synthesis of the sulphur–TiO 2 yolk–shell nanostructures The sulphur–TiO 2 yolk–shell morphology was experimentally realized as shown schematically in Fig. 2a . First, monodisperse sulphur nanoparticles were prepared using the reaction of sodium thiosulfate with hydrochloric acid ( Supplementary Fig. S1 ). The sulphur nanoparticles were then coated with TiO 2 through controlled hydrolysis of a sol-gel precursor, titanium diisopropoxide bis(acetylacetonate), in an alkaline isopropanol/aqueous solution, resulting in the formation of sulphur–TiO 2 core–shell nanoparticles ( Supplementary Fig. S2 ; the transmission electron microscopy (TEM) image was taken immediately after the electron beam was turned on to avoid sublimation of sulphur under the beam). This was followed by partial dissolution of sulphur in toluene to create an empty space between the sulphur core and the TiO 2 shell, resulting in the yolk–shell morphology. The scanning electron microscopy (SEM) image in Fig. 2b shows uniform spherical nanoparticles of ~800 nm in size. The TEM image in Fig. 2c , taken immediately after the electron beam was turned on, shows sulphur nanoparticles encapsulated within TiO 2 shells (~15 nm thick) with internal void space. Owing to the two-dimensional projection nature of TEM images, the void space will appear as either an empty area or an area of lower intensity depending on the orientation of the particles ( Fig. 2c ). The TiO 2 in the yolk–shell nanostructures were determined to be amorphous using X-ray diffraction ( Supplementary Fig. S3 ). The ability of toluene to diffuse through the TiO 2 shell to partially dissolve sulphur indicates its porous nature, which is typical of amorphous TiO 2 prepared using sol-gel methods [36] . The average pore diameter was determined to be ~3 nm using the Barrett–Joyner–Halenda method, which corresponds to a mesoporous structure. 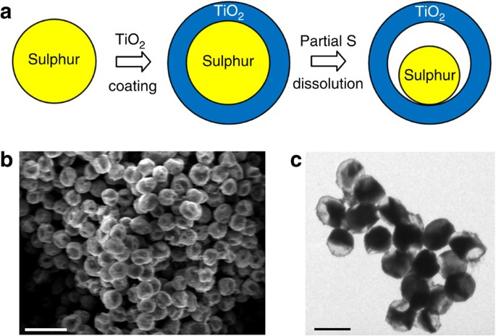Figure 2: Synthesis and characterization of sulphur–TiO2yolk–shell nanostructures. (a) Schematic of the synthetic process that involves coating of sulphur nanoparticles with TiO2to form sulphur–TiO2core–shell nanostructures, followed by partial dissolution of sulphur in toluene to achieve the yolk–shell morphology. (b) SEM image and (c) TEM image of as-synthesized sulphur–TiO2yolk–shell nanostructures. (b) Scale bar, 2 μm. (c) Scale bar, 1 μm. Through large-ensemble measurements, the average nanoparticle size and TiO2shell thickness were determined to be 800 and 15 nm, respectively. Figure 2: Synthesis and characterization of sulphur–TiO 2 yolk–shell nanostructures. ( a ) Schematic of the synthetic process that involves coating of sulphur nanoparticles with TiO 2 to form sulphur–TiO 2 core–shell nanostructures, followed by partial dissolution of sulphur in toluene to achieve the yolk–shell morphology. ( b ) SEM image and ( c ) TEM image of as-synthesized sulphur–TiO 2 yolk–shell nanostructures. ( b ) Scale bar, 2 μm. ( c ) Scale bar, 1 μm. Through large-ensemble measurements, the average nanoparticle size and TiO 2 shell thickness were determined to be 800 and 15 nm, respectively. Full size image Volume expansion in the yolk–shell nanostructures Next, we investigated the effectiveness of the yolk–shell morphology in accommodating the volume expansion of sulphur and limiting polysulphide dissolution. The sulphur–TiO 2 yolk–shell nanostructures were drop-cast onto conducting carbon paper to form working electrodes, and pouch cells were assembled using lithium foil as the counter electrode. The cells were discharged at 0.1 C (1 C=1,673 mA g −1 ) to a voltage of 1.7 V versus Li + /Li, during which a capacity of 1,110 mAh g −1 was attained ( Supplementary Fig. S4 ), and the voltage was maintained for over 20 h. The as-obtained discharge profile shows the typical two-plateau behaviour of sulphur cathodes, indicating the conversion of elemental sulphur to long-chain lithium polysulphides (Li 2 S n , 4≤ n ≤8) at ~2.3 V, and the subsequent formation of Li 2 S 2 and Li 2 S at ~2.1 V ( Supplementary Fig. S4 ) [15] , [16] , [17] , [18] . After the discharge process, the contents of the cells (cathode, anode and separator) were washed with 1,3-dioxolane (DOL) solution for further characterization. This polysulphide-containing solution was then oxidized with concentrated HNO 3 and diluted with deionized water for analysis of sulphur content using inductively coupled plasma (ICP) spectroscopy [37] . For comparison, electrode materials were also prepared using the bare sulphur and sulphur–TiO 2 core–shell nanoparticles and subject to the same treatment. There was little change in the morphology and size distribution of the sulphur–TiO 2 yolk–shell nanostructures before and after lithiation ( Fig. 3a–c ). TEM image of a lithiated yolk–shell nanostructure shows a structurally intact TiO 2 coating ( Fig. 3d ), indicating the ability of the yolk–shell design in accommodating the volume expansion of sulphur. The presence of lithiated sulphur and TiO 2 in the yolk–shell nanostructure was confirmed using energy-dispersive X-ray spectroscopy and electron energy loss spectroscopy ( Fig. 3e ). In the case of bare sulphur and sulphur–TiO 2 core–shell nanoparticles, random precipitation of irregularly shaped Li 2 S 2 and Li 2 S particles was observed on the electrodes owing to dissolution of lithium polysulphides into the electrolyte ( Supplementary Fig. S5 ) [15] , [16] , [17] , [18] . ICP analysis performed on the contents of the discharged cells showed a loss of 81 and 62% of the total sulphur mass into the electrolyte for the bare sulphur and sulphur–TiO 2 core–shell nanoparticles, respectively. In comparison, only 19% of the total sulphur mass was found to be dissolved in the electrolyte in the case of the yolk–shell nanostructures, which indicates the effectiveness of the intact TiO 2 shell in limiting polysulphide dissolution. 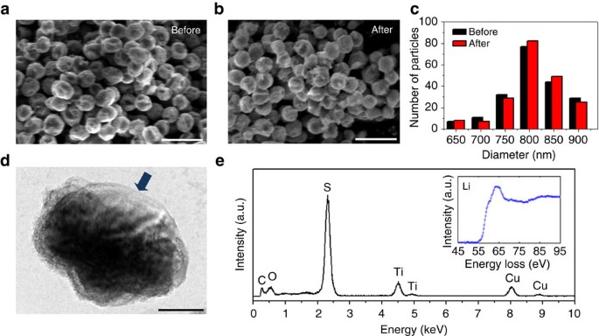Figure 3: Morphology of sulphur–TiO2yolk–shell nanostructures after lithiation. (a–c) SEM images of sulphur–TiO2yolk–shell nanostructures (a) before and (b) after lithiation and (c) their respective particle size distributions. (a,b) Scale bar, 2 μm. (d) TEM image of a sulphur–TiO2yolk–shell nanostructure after lithiation, showing the presence of an intact TiO2shell (highlighted by arrow). Scale bar, 200 nm. (e) Energy-dispersive X-ray spectrum and electron energy loss spectrum (inset) of the nanostructure in (d), showing the presence of lithiated sulphur and TiO2. The Cu peak arises owing to the use of a copper TEM grid. Figure 3: Morphology of sulphur–TiO 2 yolk–shell nanostructures after lithiation. ( a – c ) SEM images of sulphur–TiO 2 yolk–shell nanostructures ( a ) before and ( b ) after lithiation and ( c ) their respective particle size distributions. ( a , b ) Scale bar, 2 μm. ( d ) TEM image of a sulphur–TiO 2 yolk–shell nanostructure after lithiation, showing the presence of an intact TiO 2 shell (highlighted by arrow). Scale bar, 200 nm. ( e ) Energy-dispersive X-ray spectrum and electron energy loss spectrum (inset) of the nanostructure in ( d ), showing the presence of lithiated sulphur and TiO 2 . The Cu peak arises owing to the use of a copper TEM grid. Full size image Electrochemical performance To further evaluate the electrochemical cycling performance of the sulphur–TiO 2 yolk–shell nanoarchitecture, 2,032-type coin cells were fabricated. The working electrodes were prepared by mixing the yolk–shell nanostructures with conductive carbon black and polyvinylidene fluoride binder in N -methyl-2-pyrrolidinone to form a slurry, which was then coated onto aluminium foil and dried under vacuum. Using lithium foil as the counter electrode, the cells were cycled from 1.7–2.6 V versus Li + /Li. The electrolyte used was lithium bis(trifluoromethanesulfonyl)imide in 1,2-dimethoxyethane and 1,3-DOL, with LiNO 3 (1 wt%) as an additive to help passivate the surface of the lithium anode and reduce the shuttle effect [17] , [18] . Specific capacity values were calculated based on the mass of sulphur, which was determined using thermogravimetric analysis ( Supplementary Fig. S6 ). The sulphur content was found to be ~71 wt% in the yolk–shell nanostructures, accounting for ~53 wt% of the electrode mix, with a typical sulphur mass loading of 0.4–0.6 mg cm −2 . The contribution of TiO 2 to the total capacity is very small in the voltage range used in our work [38] , [39] . The sulphur–TiO 2 yolk–shell nanoarchitecture exhibited stable cycling performance over 1,000 charge/discharge cycles at 0.5 C (1 C=1,673 mA g −1 ) as displayed in Fig. 4a (see also Supplementary Fig. S7 ). After an initial discharge capacity of 1,030 mAh g −1 , the yolk–shell nanostructures achieved capacity retentions of 88, 87 and 81% at the end of 100, 200 and 500 cycles, respectively ( Fig. 4a ). Most importantly, after prolonged cycling over 1,000 cycles, the capacity retention was found to be 67%, which corresponds to a very small capacity decay of 0.033% per cycle (3.3% per 100 cycles), representing the best performance for long-cycle lithium–sulphur batteries so far. The average Coulombic efficiency over 1,000 cycles was calculated to be 98.4%, which shows little shuttle effect owing to polysulphide dissolution. In comparison, cells based on bare sulphur and sulphur–TiO 2 core–shell nanoparticles suffered from rapid capacity decay, showing capacity retentions of 48 and 66%, respectively, after only 200 cycles ( Fig. 4b ), indicating a greater degree of polysulphide dissolution into the electrolyte. 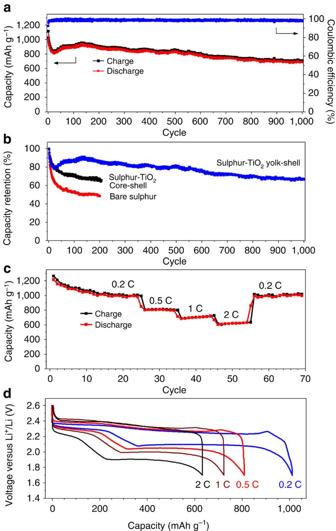Figure 4: Electrochemical performance of sulphur–TiO2yolk–shell nanostructures. (a) Charge/discharge capacity and Coulombic efficiency over 1,000 cycles at 0.5 C. (b) Capacity retention of sulphur–TiO2yolk–shell nanostructures cycled at 0.5 C, in comparison with bare sulphur and sulphur–TiO2core–shell nanoparticles. (c) Charge/discharge capacity and (d) voltage profiles of sulphur–TiO2yolk–shell nanostructures cycled at various C-rates from 0.2 to 2 C. Specific capacity values were calculated based on the mass of sulphur. Figure 4: Electrochemical performance of sulphur–TiO 2 yolk–shell nanostructures. ( a ) Charge/discharge capacity and Coulombic efficiency over 1,000 cycles at 0.5 C. ( b ) Capacity retention of sulphur–TiO 2 yolk–shell nanostructures cycled at 0.5 C, in comparison with bare sulphur and sulphur–TiO 2 core–shell nanoparticles. ( c ) Charge/discharge capacity and ( d ) voltage profiles of sulphur–TiO 2 yolk–shell nanostructures cycled at various C-rates from 0.2 to 2 C. Specific capacity values were calculated based on the mass of sulphur. Full size image Next, the sulphur–TiO 2 yolk–shell nanostructures were subject to cycling at various C-rates to evaluate their robustness ( Fig. 4c ). After an initial discharge capacity of 1,215 mAh g −1 at 0.2 C, the capacity was found to stabilize at 1,010 mAh g −1 . Further cycling at 0.5, 1 and 2 C showed high reversible capacities of 810, 725 and 630 mAh g −1 , respectively ( Fig. 4c ). When the C-rate was switched abruptly from 2 to 0.2 C again, the original capacity was largely recovered ( Fig. 4c ), indicating robustness and stability of the cathode material. Moreover, there was little change in the thickness of the cathode before and after 70 cycles at these various C-rates ( Supplementary Fig. S8 ), which further confirms the ability of the yolk–shell nanostructures in accommodating the volume expansion of sulphur. There are two important characteristics of such a yolk–shell design that imparts the sulphur–TiO 2 nanostructures with stable cycling performance over 1,000 charge/discharge cycles. First, sufficient empty space was present to allow for volume expansion of sulphur. Using image processing software on the yolk–shell nanostructures ( Fig. 2c ), sulphur was determined to occupy ~62% of the volume within the TiO 2 shell, which corresponds to 38% internal void space. This value is supported by thermogravimetric analysis of the relative wt% of sulphur versus TiO 2 ( Supplementary Fig. S6 ), from which the volume of empty space in the yolk–shell nanostructures was estimated to be 37%. This volume of void space can accommodate ~60% volume expansion of the sulphur present within the shell, allowing for 1,250 mAh g −1 , that is, 75% of the maximum theoretical capacity of sulphur, to be utilized (assuming volume expansion is linearly dependent on the degree of lithiation). Experimentally, we have been able to achieve a maximum discharge capacity of 1,215 mAh g −1 ( Fig. 4c ), therefore there is sufficient void space for volume expansion without causing the shell to crack and fracture. Second, the intact TiO 2 shell, with its small pore size of ~3 nm, was effective in minimizing polysulphide dissolution. Mesoporous structures, such as those based on carbon, have been shown to help trap polysulphides owing to their small pore sizes (~3 nm) [20] , [27] . Moreover, metal oxides such as TiO 2 possess hydrophilic Ti–O groups and surface hydroxyl groups, which are known to bind favourably with polysulphide anions, hence further limiting the extent of polysulphide dissolution [21] , [40] . In conclusion, we have demonstrated for the first time, the design of a sulphur–TiO 2 yolk–shell nanoarchitecture for long cycling capability over 1,000 charge/discharge cycles, with a capacity decay as small as 0.033% per cycle. Compared with its bare sulphur and sulphur–TiO 2 core–shell counterparts, the yolk–shell nanostructures exhibited the highest capacity retention owing to the presence of internal void space to accommodate the volume expansion of sulphur during lithiation, resulting in an intact shell to minimize polysulphide dissolution. Insight gained from this work can be applied to other high-capacity anode and cathode material systems, especially those that undergo large volumetric expansion, providing new avenues for the future development of high-performance rechargeable batteries. Synthesis of sulphur–TiO 2 yolk–shell nanostructures First, sulphur nanoparticles were synthesized by adding concentrated HCl (0.8 ml, 10 M) to an aqueous solution of Na 2 S 2 O 3 (100 ml, 0.04 M) containing a low concentration of polyvinylpyrrolidone (PVP, M w ~55,000, 0.02 wt%; we note that at much higher PVP concentrations, hollow sulphur particles are formed instead). After reaction for 2 h, the sulphur nanoparticles (100 ml) were washed by centrifugation and redispersed into an aqueous solution of PVP (20 ml, 0.05 wt%). For TiO 2 coating, the solution of sulphur nanoparticles (20 ml) was mixed with isopropanol (80 ml) and concentrated ammonia (2 ml, 28 wt%). Titanium diisopropoxide bis(acetylacetonate) (50 ml, 0.01 M in isopropanol) was then added in five portions (5 × 10 ml) at half hour intervals. After reaction for 4 h, the solution of sulphur–TiO 2 core–shell nanoparticles was washed by centrifugation to remove freely hydrolysed TiO 2 , followed by redispersion into deionized water (20 ml). To prepare the sulphur–TiO 2 yolk–shell nanostructures, the solution of core–shell particles (20 ml) was stirred with isopropanol (20 ml) and toluene (0.4 ml) for 4 h to achieve partial dissolution of sulphur. The as-synthesized sulphur–TiO 2 yolk–shell nanostructures were then recovered using centrifugation and dried under vacuum overnight. Characterization SEM and TEM images were taken using a FEI XL30 Sirion SEM (accelerating voltage 5 kV) and a FEI Tecnai G2 F20 X-TWIN (accelerating voltage 200 kV), respectively. Elemental analysis was performed using energy-dispersive X-ray spectroscopy and electron energy loss spectroscopy equipped in the TEM. X-ray diffraction patterns were obtained on a PANalytical X’Pert Diffractometer using Cu Kα radiation. Thermogravimetric analysis was carried out using a Netzsch STA 449 at a heating rate of 2 °C min −1 under argon atmosphere. ICP optical emission spectroscopy was performed using a Thermo Scientific ICAP 6300 Duo View Spectrometer. Nitrogen adsorption data were collected on a Micromeritics ASAP 2020 Analyser after degassing at 180 °C for 12 h. Electrochemical measurements To prepare the working electrodes, the various sulphur-based materials were mixed with carbon black (Super P) and polyvinylidene fluoride binder (75:15:10 by weight) in N -methyl-2-pyrrolidinone to form a slurry. This slurry was then coated onto aluminium foil using doctor blade and dried under vacuum to form the working electrode. 2032-type coin cells were assembled in an argon-filled glove box using lithium foil as the counter electrode. The electrolyte used was a freshly prepared solution of lithium bis(trifluoromethanesulfonyl)imide (1 M) in 1:1 v/v 1,2-dimethoxyethane and 1,3-DOL containing LiNO 3 (1 wt%). Galvanostatic cycling was carried out using a 96-channel battery tester (Arbin Instruments) from 1.7–2.6 V versus Li + /Li. Specific capacity values were calculated based on the mass of sulphur in the samples, which was determined using thermogravimetric analysis ( Supplementary Fig. S6 ). The sulphur content was found to be ~71 wt% in the yolk–shell nanostructures, accounting for ~53 wt% of the electrode mix, with a typical sulphur mass loading of 0.4–0.6 mg cm −2 . How to cite this article: Seh, Z. W. et al . Sulphur–TiO 2 yolk–shell nanoarchitecture with internal void space for long-cycle lithium–sulphur batteries. Nat. Commun. 4:1331 doi: 10.1038/ncomms2327 (2013).